A CLASP-modulated cell edge barrier mechanism drives cell-wide cortical microtubule organization in Arabidopsis It is well known that the parallel order of microtubules in the plant cell cortex defines the direction of cell expansion, yet it remains unclear how microtubule orientation is controlled, especially on a cell-wide basis. Here we show through 4D imaging and computational modelling that plant cell polyhedral geometry provides spatial input that determines array orientation and heterogeneity. Microtubules depolymerize when encountering sharp cell edges head-on, whereas those oriented parallel to those sharp edges remain. Edge-induced microtubule depolymerization, however, is overcome by the microtubule-associated protein CLASP, which accumulates at specific cell edges, enables microtubule growth around sharp edges and promotes formation of microtubule bundles that span adjacent cell faces. By computationally modelling dynamic 'microtubules on a cube' with edges differentially permissive to microtubule passage, we show that the CLASP-edge complex is a 'tuneable' microtubule organizer, with the inherent flexibility to generate the numerous cortical array patterns observed in nature. Plant tissues contain cells that are polyhedral in shape. The sharp edges marking the boundaries between adjacent cell faces present an interesting challenge to relatively rigid microtubules (MTs), which cover much of the cell cortex. By organizing into parallel arrays, cortical MTs affect cell wall properties, promoting expansion at right angles to their predominant orientation. The parallel nature and orientation of cortical MT arrays in plant cells raise three tantalizing questions: First, how do MTs become aligned parallel to each other? Second, in the absence of clear spatial input from a central organizer (such as centrosomes), what determines whether an array will be oriented transverse or longitudinal relative to the cell axis? And finally, how is the orientation of cortical arrays coordinated between different cell faces [1] ? Live imaging studies over the past decade have clarified our understanding of how MTs form parallel arrays. Following the in vivo characterization of MT dynamic instability parameters by Shaw et al . [2] , several papers have focused on how interactions between MTs facilitate self-organization into large-scale MT arrays [3] , [4] , [5] . These self-organizational mechanisms include bundling of MTs on encounter at small contact angles [6] , MT catastrophe on steep angle collision with another MT [6] , MT severing at cross over points [7] , MT branch-and-release from pre-existing MTs [8] , [9] , co-parallel MT nucleation within bundles [10] , [11] , and MT-detachment-based bundle formation [11] . In addition to these small-scale self-organizational mechanisms, large-scale behaviours such as rotary movements of MT arrays [12] and domains of homogeneous MT growth orientation [12] , [13] have also been described. Recent computational modelling studies have supported these ideas by using empirically measured MT dynamic parameters to simulate self-organized, parallel arrays [14] , [15] , [16] . How array orientation direction is determined, in the absence of a central organizer, is less clear. It has long been predicted and recently confirmed by imaging shoot apical meristems that MTs align according to major stress lines [17] , yet, a mechanism for such alignment remains to be identified. Mutations in genes encoding various MT-associated proteins and tubulins generate cortical arrays that are sometimes abnormally tilted from their typical transverse arrangement in elongating cells [18] , [19] , suggesting that modulation of intrinsic MT assembly dynamics by MT-associated proteins is involved. How the specific handedness of MT array tilt is achieved in these mutants, however, is unknown and computational modelling using the dynamic MT parameters measured in these mutants fails to recapitulate the phenotypes of these mutants [16] . Cytoplasmic streaming can flow-orient microtubules, especially when they are partially detached from the cortex [11] , [20] , [21] , [22] , but this myosin motor-dependent mechanism is likely to be only a minor contributor to overall MT orientation. Elongating cells display distinct orientations of MTs on different cell faces, with transverse arrays typical along the growing longitudinal faces and radially arranged arrays along the non-expanding transverse faces [1] , [23] , [24] , [25] . It has been hypothesized that an asymmetric distribution of MT catastrophe factors at cell ends could contribute to the formation of transverse MT arrays on the longitudinal faces [26] . A non-biochemical mechanism has also been suggested by in vitro experiments of MT assembly in microfabricated chambers [27] , which demonstrated that when MT lengths exceed cell circumference, a longitudinal orientation is energetically preferred, as this orientation confers less bending on MTs. More recently, computer simulations of cortical MT arrays incorporating self-organizational mechanisms in the model predicted that catastrophe-inducing boundaries on two opposing cell faces are sufficient to form MT arrays with a net transverse orientation [15] , [16] , [28] . Here we combine live cell imaging and computational modelling to demonstrate that by inducing MT catastrophe, cell edges influence cell-wide MT organization, and that the protein CLASP modulates this edge effect to generate array complexity during cell expansion and division. CLASP localizes to cell edges The nomenclature used in this article is as follows. Each cell is composed of faces and edges ( Fig. 1a ). Periclinal faces are parallel to the organ surface, and anticlinal faces are perpendicular to it. To distinguish the two types of anticlinal faces in roots, we use transverse (cross-walls), and radial (sidewalls). For edge nomenclature in roots, edges are named by their orientation with respect to the root axis: longitudinal, transverse, and radial. In leaf epidermal cells, the edges are termed periclinal or anticlinal. 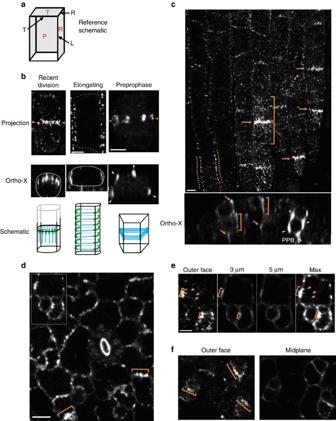Figure 1: CLASP protein accumulates at cell edges in unexpanded cells. (a) Schematic of edge and face nomenclature. Cell faces indicated in red text, cell edges in black text. L, longitudinal; P, periclinal; R, radial; T, transverse. (b) Root cells showing differential cell edge accumulation of GFP–CLASP at three different stages: recently divided, expanding, and preprophase cells. Cells are shown as maximum Z projections, and orthogonal views, and are accompanied by reference schematics (MTs, blue lines; GFP–CLASP, green). (c) Root tip cells exhibit strong GFP–CLASP expression and show non-uniform accumulation of GFP–CLASP around the cell edges. Shown is a confocal Z-projection through the outer half of the lateral root cap cells covering the root division zone. Arrows indicate GFP–CLASP enrichment at the shared wall between recently divided cells. Brackets indicate two adjacent cells. Dotted lines indicate GFP–CLASP enrichment along longitudinal edges of expanding cells. Bottom panel shows an X-orthogonal view through a GFP–CLASP expressing root tip. Arrows indicate GFP–CLASP on longitudinal edges. Brackets indicate enrichment covering the entire radial cell faces in smaller cells, in contrast to the edge-specific accumulation in larger cells. (d) Unexpanded leaf epidermal cells. Brackets indicate domains of GFP–CLASP accumulation at newly formed cross-walls. Image is a maximum Z-projection of a confocal stack from the leaf surface into the epidermal midplane. (e) Cell from inset in (d) showing single optical planes at three depths, and max Z projection. Brackets indicate GFP–CLASP edge domains. Arrows indicate MT lattice labelling on periclinal face. (f) Examples of strong GFP–CLASP enrichment at recently formed cross-walls of leaf epidermal cells. Single optical sections at the outer face and cellular midplane. Brackets indicate GFP–CLASP edge domains. The scale bars represent 5 μm. Figure 1: CLASP protein accumulates at cell edges in unexpanded cells. ( a ) Schematic of edge and face nomenclature. Cell faces indicated in red text, cell edges in black text. L, longitudinal; P, periclinal; R, radial; T, transverse. ( b ) Root cells showing differential cell edge accumulation of GFP–CLASP at three different stages: recently divided, expanding, and preprophase cells. Cells are shown as maximum Z projections, and orthogonal views, and are accompanied by reference schematics (MTs, blue lines; GFP–CLASP, green). ( c ) Root tip cells exhibit strong GFP–CLASP expression and show non-uniform accumulation of GFP–CLASP around the cell edges. Shown is a confocal Z-projection through the outer half of the lateral root cap cells covering the root division zone. Arrows indicate GFP–CLASP enrichment at the shared wall between recently divided cells. Brackets indicate two adjacent cells. Dotted lines indicate GFP–CLASP enrichment along longitudinal edges of expanding cells. Bottom panel shows an X-orthogonal view through a GFP–CLASP expressing root tip. Arrows indicate GFP–CLASP on longitudinal edges. Brackets indicate enrichment covering the entire radial cell faces in smaller cells, in contrast to the edge-specific accumulation in larger cells. ( d ) Unexpanded leaf epidermal cells. Brackets indicate domains of GFP–CLASP accumulation at newly formed cross-walls. Image is a maximum Z-projection of a confocal stack from the leaf surface into the epidermal midplane. ( e ) Cell from inset in (d) showing single optical planes at three depths, and max Z projection. Brackets indicate GFP–CLASP edge domains. Arrows indicate MT lattice labelling on periclinal face. ( f ) Examples of strong GFP–CLASP enrichment at recently formed cross-walls of leaf epidermal cells. Single optical sections at the outer face and cellular midplane. Brackets indicate GFP–CLASP edge domains. The scale bars represent 5 μm. Full size image To follow CLASP's distribution at physiologically relevant expression levels, we used the CLASP gene's endogenous promoter to drive expression of a GFP–CLASP fusion protein, which in the clasp-1 null mutant fully complements the clasp-1 phenotype ( Supplementary Fig. S1 ). CLASP expression, as indicated by fluorescence intensity, was highest in regions of active cell division and cell expansion, particularly in root tips and the expanding leaf epidermis. Expanded, vacuolated cells, in which CLASP's distribution along MTs was previously studied [29] , [30] , contained comparatively little GFP–CLASP. In newly formed cells of the root division zone, GFP–CLASP was enriched along the transverse and/or longitudinal edges in a stage of development-dependent manner, with a weaker intensity associated with MTs on the outer periclinal face ( Fig. 1b,c ). CLASP edge distribution was non-uniform, forming distinct domains that were persistent over tens of minutes, yet exhibited rapid turnover of CLASP molecules, as evidenced by GFP–CLASP's photobleach recovery in 10–20 seconds ( Supplementary Fig. S2a–c ). In recently formed root cells (5–10 min after phragmoplast disappearance), CLASP was enriched along the outer transverse edge ( Fig. 1b,c ). The signal intensity and immobility of GFP–CLASP was highest during this early stage. Edge distribution was particularly prominent in cells containing preprophase bands (PPBs), in which GFP–CLASP accumulated only at edges intersected by the band ( Fig. 1b,c ). CLASP levels gradually tapered off in the elongation zone, and GFP–CLASP became distributed along the longitudinal edges ( Fig. 1b,c ). In elongating root cells with smaller diameters (particularly lateral root cap cells), GFP–CLASP often covered entire radial faces ( Fig. 1b,c ). A mix of these GFP–CLASP distributions was found in the transition between the division and elongation zones. In the polyhedral cells of the unexpanded leaf epidermis, GFP–CLASP accumulated soon after cell division at the outer edge of the newly formed cross-wall, as in roots ( Fig. 1d–f ; Supplementary Movie 1 ). Along older edges, GFP–CLASP formed patches of varying sizes, often with associated MT labelling along the outer periclinal face ( Fig. 1d–f ). Coexpressing GFP–CLASP and Ubiquitin1 promoter-driven RFP–βTubulin6 (RFP–TUB6) identified MT bundles intersecting cell edges at CLASP edge domains and extending into the neighbouring face, forming transfacial bundles (TBs; Fig. 2 ; Supplementary Movie 2 ). Like GFP–CLASP, TBs were positionally persistent (mean persistence time 19.0±5.4 min, n =45 cells, n =79 TBs in root division zone cells), but contained dynamic MTs, as evidenced by observing MT plus-end growth with EB1b–GFP ( Supplementary Fig. S2d,e ). GFP–CLASP domains resemble arc-shaped elements that curve around the cell edge in association with TBs ( Fig. 2a,b ). TB-like structures have previously been observed in electron micrographs from root tip cells of the fern Azolla [31] . 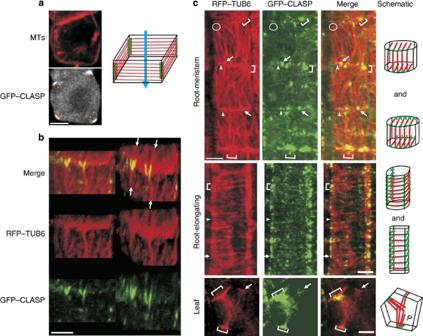Figure 2: Transfacial MT bundles intersect GFP–CLASP edge domains. (a) A GFP–CLASP-expressing division zone cell (with transverse MTs) fixed and mounted (seeMethods) such that it is viewed through the top-bottom axis. Arrowheads indicate GFP–CLASP edge domains. Co-staining with anti-tubulin (MTs, red) shows uniform MT distribution around the cell sides. Reference schematic depicts MTs in red, CLASP in green. (b) Transfacial MT bundles (TBs) intersect cell edges at GFP–CLASP domains. Maximum 3D reconstructions at 0 and 30 degrees (X-axis) enable simultaneous viewing of transverse and periclinal faces. Shown is a UBQ1:RFP–TUB6 (red) and GFP–CLASP (green) coexpressing root meristematic cell. (c) Codistribution of UBQ1:RFP–TUB6 (red) and GFP–CLASP (green) in young root and leaf cells. Symbols indicate various sizes of TB/GFP–CLASP edge intersections (Arrowheads=single MTs/small bundles; arrows=single moderate bundles; brackets=convergence of multiple bundles at intense GFP–CLASP domains; circles=passage of longitudinal TBs around rounded region of transverse edge, and associated lack of noticeable GFP–CLASP signal). The top panel shows cells from the division zone, middle panel shows a cell from the early elongation zone, bottom panel shows an unexpanded leaf cell. In the leaf images, the large TBs appear oversaturated due to the strong contrasting required to reveal the smaller TBs against the background of autofluorescent vacuolar anthocyanins. The scale bars represent 5 μm. Figure 2: Transfacial MT bundles intersect GFP–CLASP edge domains. ( a ) A GFP–CLASP-expressing division zone cell (with transverse MTs) fixed and mounted (see Methods ) such that it is viewed through the top-bottom axis. Arrowheads indicate GFP–CLASP edge domains. Co-staining with anti-tubulin (MTs, red) shows uniform MT distribution around the cell sides. Reference schematic depicts MTs in red, CLASP in green. ( b ) Transfacial MT bundles (TBs) intersect cell edges at GFP–CLASP domains. Maximum 3D reconstructions at 0 and 30 degrees (X-axis) enable simultaneous viewing of transverse and periclinal faces. Shown is a UBQ1:RFP–TUB6 (red) and GFP–CLASP (green) coexpressing root meristematic cell. ( c ) Codistribution of UBQ1:RFP–TUB6 (red) and GFP–CLASP (green) in young root and leaf cells. Symbols indicate various sizes of TB/GFP–CLASP edge intersections (Arrowheads=single MTs/small bundles; arrows=single moderate bundles; brackets=convergence of multiple bundles at intense GFP–CLASP domains; circles=passage of longitudinal TBs around rounded region of transverse edge, and associated lack of noticeable GFP–CLASP signal). The top panel shows cells from the division zone, middle panel shows a cell from the early elongation zone, bottom panel shows an unexpanded leaf cell. In the leaf images, the large TBs appear oversaturated due to the strong contrasting required to reveal the smaller TBs against the background of autofluorescent vacuolar anthocyanins. The scale bars represent 5 μm. Full size image CLASP edge domain distribution varied with cell type and age, being generally enriched at the edges intersected by MTs in the dominant orientation ( Fig. 2c ). The size and signal intensity of GFP–CLASP edge domains correlated with the size of the intersecting MT bundle: small GFP–CLASP spots associated with small TBs (arrowheads), moderate spots associated with moderate TBs (arrows), and the largest GFP–CLASP domains were at edge regions where multiple TBs converged (brackets; Fig. 2c ). Partial Z-projections, such as the 3 μm maximum z-stacks shown in Figure 1c, do not show the complete population of edge-associated GFP–CLASP, as the GFP–CLASP signal was sometimes confined to fewer optical planes than the TBs, whose curved linear structures extended across the cell faces. To quantify the association of GFP–CLASP with the RFP–TUB6-labelled TBs, we therefore manually scrolled through merged-colour optical series (an example of one such z-stack is provided in Supplementary Movie 2 ). In unexpanded leaf epidermal cells, GFP–CLASP accumulated in strong patches intersected by several TBs, most likely corresponding to the prominent bands of MT bundles associated with neck formation during epidermal cell interdigitation [32] , [33] ( Fig. 2c ). Transfacial bundle-CLASP intersections are specific to sharp edges In seeking to understand the relationship between CLASP's distribution to particular cell edges and the formation of TBs, we compared the curvature of edges rich in GFP–CLASP fluorescence with those edges lacking it. In the root division zone, the transverse and radial edges of epidermal cells are consistently sharp (being derived from recent cell division), whereas longitudinal edges are rounded ( Fig. 3a–c ). In these cells, GFP–CLASP showed enrichment on the transverse edges, and was intersected by TBs in 96.4±0.3% of cases ( Fig. 3d,e ; n =42 cells). Along the semi-rounded longitudinal edges, GFP–CLASP was faint to non-detectable where TBs could be observed, being of similar intensity to that of the weak MT lattice labelling seen on the outer periclinal face, and roughly threefold less than that along the sharp transverse edges ( Fig. 3f ). The few instances of TBs crossing transverse edges without associated GFP–CLASP included the rounded edges at the site of cell separation along the outer perimeter of the transverse walls ( Fig. 2c , circled region). Radial edges are, like transverse edges, very sharp, yet GFP–CLASP and TBs along radial edges were undetectable, thereby excluding a generalized preference for all sharp edges. GFP–CLASP signal intensity was also greatest along the recently formed sharp cell edges of leaf epidermal cells, in which edge curvature is variable around the perimeter of the outer periclinal face ( Fig. 3g,h ). Taken together, these data indicate an enrichment of CLASP at specific sharp edges, and, importantly, exclude the possibility that CLASP edge accumulation is merely a coincidental outcome of MT bundles bypassing edges in general. 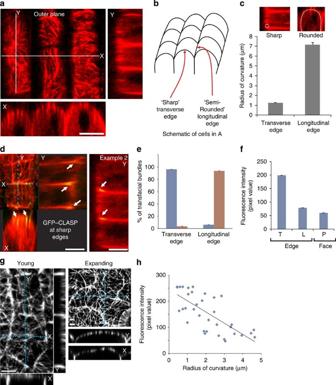Figure 3: CLASP is enriched at select sharp edges. (a) Wild-type root epidermal division zone cells visualized using RFP–TUB6. Shown are the outer periclinal cell faces (single optical section), and X and Y orthogonal views corresponding to the cross. (b) Schematic of cells in (a), depicting sharp transverse edges, and semi-rounded longitudinal edges. (c) Measurements of radius of curvature for wild-type root epidermal division zone cells. Data are taken from 85 wild-type cells, measuring 165 transverse edges, and 154 longitudinal edges. Data are means±s.e.m. (d) Wild-type root epidermal division zone cells coexpressing GFP–CLASP and RFP–TUB6. Single optical plane, X and Y orthogonal views are shown. Arrows indicate GFP–CLASP transverse edge accumulation. (e) Percentage of TBs intersecting GFP–CLASP edge domains in root epidermal division zone cells, comparing TBs that cross sharp (transverse) edges with semirounded (longitudinal) edges. Blue bars indicate TBs intersecting GFP–CLASP domains, red bars indicate TBs not intersecting GFP–CLASP edge domains (n=42 cells, 241 sharp edge TBs, 129 round edge TBs). (f) GFP–CLASP is enriched at transverse edges in root epidermal division zone cells. Single pixel intensity values at GFP–CLASP maxima (n=88 transverse edges, 87 longitudinal edges). T=transverse edge; L=Longitudinal edge; P=outer periclinal face. (g,h) GFP–CLASP enrichment at sharp edges correlates with edge curvature in variable curvature leaf epidermal cells. (g) Young and expanding cells shown in max Z projection and X and Y orthogonal views. Young cells contain sharper edges than expanding cells. (h) GFP–CLASP edge signal intensity correlates inversely with radius of curvature. (n=36 cells). The scale bars represent 5 μm. Figure 3: CLASP is enriched at select sharp edges. ( a ) Wild-type root epidermal division zone cells visualized using RFP–TUB6. Shown are the outer periclinal cell faces (single optical section), and X and Y orthogonal views corresponding to the cross. ( b ) Schematic of cells in ( a ), depicting sharp transverse edges, and semi-rounded longitudinal edges. ( c ) Measurements of radius of curvature for wild-type root epidermal division zone cells. Data are taken from 85 wild-type cells, measuring 165 transverse edges, and 154 longitudinal edges. Data are means±s.e.m. ( d ) Wild-type root epidermal division zone cells coexpressing GFP–CLASP and RFP–TUB6. Single optical plane, X and Y orthogonal views are shown. Arrows indicate GFP–CLASP transverse edge accumulation. ( e ) Percentage of TBs intersecting GFP–CLASP edge domains in root epidermal division zone cells, comparing TBs that cross sharp (transverse) edges with semirounded (longitudinal) edges. Blue bars indicate TBs intersecting GFP–CLASP domains, red bars indicate TBs not intersecting GFP–CLASP edge domains ( n =42 cells, 241 sharp edge TBs, 129 round edge TBs). ( f ) GFP–CLASP is enriched at transverse edges in root epidermal division zone cells. Single pixel intensity values at GFP–CLASP maxima ( n =88 transverse edges, 87 longitudinal edges). T=transverse edge; L=Longitudinal edge; P=outer periclinal face. ( g , h ) GFP–CLASP enrichment at sharp edges correlates with edge curvature in variable curvature leaf epidermal cells. ( g ) Young and expanding cells shown in max Z projection and X and Y orthogonal views. Young cells contain sharper edges than expanding cells. ( h ) GFP–CLASP edge signal intensity correlates inversely with radius of curvature. ( n =36 cells). The scale bars represent 5 μm. Full size image Microtubules orient parallel to sharp edges lacking CLASP CLASP's strong enrichment along sharp cell edges where TBs intersect suggests that CLASP acts to locally stabilize MTs in these edge regions. To test this possibility, we compared MT organization in clasp-1 null mutants and wild-type plants. 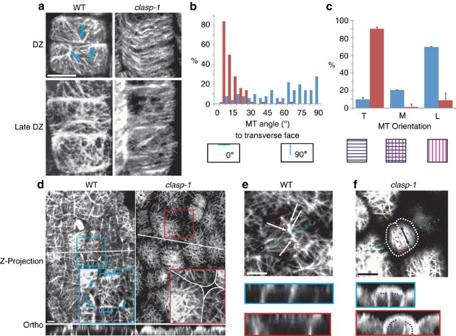Figure 4: MTs orient parallel to sharp edges in the absence of CLASP. (a) Root tip epidermal cells from division zone (DZ) and early elongation zone (EZ) in wild type andclasp-1mutants. Images are single optical sections. MTs are visualized using anti-tubulin immunofluorescence. We excluded the possibility that the lack of observable CTBs inclasp-1is due to mistaking elongating cells from true division zone cells inclasp-1, which contains smaller meristems. Examining MT patterns in 384 cells from 13clasp-1roots (a sample size sufficient to capture all cell cycle stages) failed to show any incidence of TBs at transverse edges and very few non-transverse arrays. (b) Quantification of MT angles relative to sharp (transverse) edges in wild-type (blue bars) andclasp-1(red bars) root epidermal division zone cells. (n=40 cells, 200 MTs). (c) Quantification of relative abundance of MT arrays according to orientation in division zones of wild-type (blue bars) andclasp-1(red bars) roots. Arrays were labelled using anti-tubulin immunofluorescence and classified cell by cell as transverse (T), mixed (M), and longitudinal (L). Forclasp-1,n=384 cells, 13 roots. For wild type,n=306 cells, 11 roots. Data are mean percentages±s.e. (d) Young leaf epidermal cells of wild type andclasp-1. Shown are Z-projections that extend into the cell midplane. MTs were visualized using GFP–MBD. Brackets indicate TBs in insets. Lines indicate orthogonal views. (e,f) Leaf epidermal cells from wild type andclasp-1. Shown for each are single optical planes, and orthogonal views (indicated by dotted lines). (e) Wild type. Arrows indicate TBs intersecting at right angles in wild type. (f)clasp-1. Cell indicated by white dotted outline. Double arrows indicate MT orientation. The scale bars represent 5 μm. As shown in Figure 4 , clasp-1 mutants displayed a marked reduction in TBs in both root tips and young leaves. Importantly, TBs were absent at sharp cell edges but could still be observed at rounded edges. We therefore define TBs that cross sharp, CLASP-populated edges as CLASP-mediated transfacial bundles (CTBs). Figure 4: MTs orient parallel to sharp edges in the absence of CLASP. ( a ) Root tip epidermal cells from division zone (DZ) and early elongation zone (EZ) in wild type and clasp-1 mutants. Images are single optical sections. MTs are visualized using anti-tubulin immunofluorescence. We excluded the possibility that the lack of observable CTBs in clasp-1 is due to mistaking elongating cells from true division zone cells in clasp-1 , which contains smaller meristems. Examining MT patterns in 384 cells from 13 clasp-1 roots (a sample size sufficient to capture all cell cycle stages) failed to show any incidence of TBs at transverse edges and very few non-transverse arrays. ( b ) Quantification of MT angles relative to sharp (transverse) edges in wild-type (blue bars) and clasp-1 (red bars) root epidermal division zone cells. ( n =40 cells, 200 MTs). ( c ) Quantification of relative abundance of MT arrays according to orientation in division zones of wild-type (blue bars) and clasp-1 (red bars) roots. Arrays were labelled using anti-tubulin immunofluorescence and classified cell by cell as transverse (T), mixed (M), and longitudinal (L). For clasp-1 , n =384 cells, 13 roots. For wild type, n =306 cells, 11 roots. Data are mean percentages±s.e. ( d ) Young leaf epidermal cells of wild type and clasp-1 . Shown are Z-projections that extend into the cell midplane. MTs were visualized using GFP–MBD. Brackets indicate TBs in insets. Lines indicate orthogonal views. ( e,f ) Leaf epidermal cells from wild type and clasp-1 . Shown for each are single optical planes, and orthogonal views (indicated by dotted lines). ( e ) Wild type. Arrows indicate TBs intersecting at right angles in wild type. ( f ) clasp-1 . Cell indicated by white dotted outline. Double arrows indicate MT orientation. The scale bars represent 5 μm. Full size image In recently divided wild-type root division zone cells, CTBs intersecting the sharp transverse edges define a dominant longitudinal MT orientation or contribute to a mixed MT organization [24] on the outer periclinal face ( Fig. 4a ). In contrast, MTs in clasp-1 root tips were consistently oriented parallel to the sharp transverse edges ( Fig. 4a,b ), resulting in a preponderance of transverse arrays ( Fig. 4c ). The lack of TBs at the recently formed cell edges in clasp-1 roots was also evident by the greatly diminished MT-specific fluorescence at the focal midplane in comparison to wild-type cells ( Supplementary Fig. S3a–e ). In young leaf epidermal cells of clasp-1 mutants, the absence of CTBs was associated with an apparently random distribution of MTs at the periclinal face, with MTs only occasionally extending around the edges into the anticlinal faces ( Fig. 4d ). Taking advantage of the fact that the most recently divided leaf epidermal cells contain both sharp, newly-formed edges and rounded older edges, we confirmed that CTBs intersected at right angles the newly formed sharp edges in wild-type cells ( Fig. 4e ). By contrast, MTs in clasp-1 mutants were oriented parallel to these sharp edges but could extend onto the anticlinal face at the rounded edges ( Fig. 4f ). Thus, CLASP is required for CTBs to intersect the newly formed edges in both root and leaf epidermal cells. Clasp-1 leaf epidermal cells exhibited premature outward bulging, which resulted in more rounded periclinal edges ( Fig. 4d–f ; Supplementary Fig. S4a ). Similarly, in roots, transverse edges were more rounded in clasp-1 epidermal and lateral root cap cells compared with wild type ( Supplementary Fig. S4b ). CLASP is thus required to maintain sharp cell edges in leaf and root epidermal cells. Sharp edges induce MT buckling and catastrophe On the basis of the above correlation between edge curvature and MT orientation, we hypothesized that sharp cell edges present a physical barrier to MTs. MT depolymerization and buckling are known to occur in response to the axial compression resulting from polymerization against an obstruction [7] , [34] . Indeed, we observed that, in young wild-type leaf epidermal cells, MTs encountering the sharp periclinal cell edges underwent catastrophe at the point of edge encounter ( Fig. 5a ; Supplementary Movie 3 ). MTs encountering these edges often buckled before depolymerization, which is suggestive of a growth-impeding physical obstruction [7] , [34] ( Fig. 5b ; Supplementary Movie 4 ). Sharp edge-induced MT buckling was more obvious in the clasp-1 mutant, perhaps due to the weakened cortical attachment of MTs, which allows greater lateral mobility [11] , [34] . ( Fig. 5c ; Supplementary Movie 5 ). 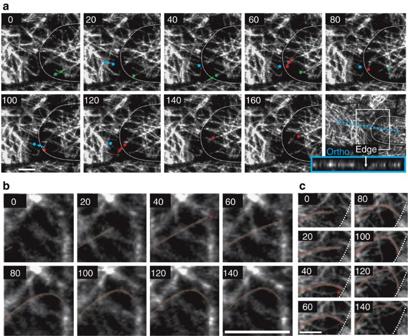Figure 5: Sharp edges induce MT catastrophe and buckling. (a) Time series from wild-type early elongating petiole cells. The time sequence is taken from the boxed region in the bottom right panel CTB-free cell ends characteristic of elongating cells with transverse arrays. Dots indicate MT plus-ends, dotted lines indicate cell edges. Arrows indicate directionality of growth or shortening in each case. Orthogonal view corresponds to the blue dotted line, and illustrates degree of edge curvature. (b) MT buckling on edge encounter in a wild-type leaf epidermal cell. Asterisk indicates initial edge encounter. (c) MT buckling on edge encounter in aclasp-1leaf epidermal cell. Asterisk denotes initial edge encounter. The MT is released near the end of the sequence. The scale bars represent 5 μm. Times are in seconds. Figure 5: Sharp edges induce MT catastrophe and buckling. ( a ) Time series from wild-type early elongating petiole cells. The time sequence is taken from the boxed region in the bottom right panel CTB-free cell ends characteristic of elongating cells with transverse arrays. Dots indicate MT plus-ends, dotted lines indicate cell edges. Arrows indicate directionality of growth or shortening in each case. Orthogonal view corresponds to the blue dotted line, and illustrates degree of edge curvature. ( b ) MT buckling on edge encounter in a wild-type leaf epidermal cell. Asterisk indicates initial edge encounter. ( c ) MT buckling on edge encounter in a clasp-1 leaf epidermal cell. Asterisk denotes initial edge encounter. The MT is released near the end of the sequence. The scale bars represent 5 μm. Times are in seconds. Full size image CLASP mitigates the barrier effect of sharp cell edges On the basis of CLASP's co-localization with CTBs at cell edges and its requirement for CTB formation, we hypothesized that CLASP acts to locally stabilize the plus-ends of MTs encountering cell edges, allowing them to continue growth around the edge. To test this hypothesis, we first imaged young wild-type leaf epidermal cells and compared the frequency of catastrophe on edge encounter in regions occupied by CTBs (that is, CLASP edge domains) with regions lacking these bundles (CTB-free; as indicated in Fig. 6a ). There was a striking difference in the behaviour of MTs in these two regions. MTs encountering CTB-free edge domains underwent catastrophe 84±2% of the time ( n =100 MTs, 23 cells), whereas the catastrophe frequency at CTB edge domains was only 9.7±8.5% ( n =72 MTs, 15 cells). 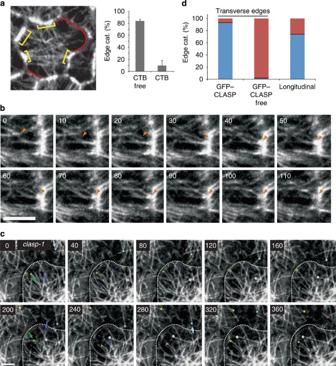Figure 6: CLASP mitigates the barrier effect of sharp cell edges. (a) Percentage of MTs that undergo catastrophe on encounter of CTB versus CTB-free cell edges in young leaf epidermal cells. (n=38 cells, 172 MTs; bars are mean percentages±s.e). Yellow brackets indicate CTBs, Red lines indicate CTB-free domains (using CTBs as proxies for GFP–CLASP domains.) (b) MT persistence on encountering a CTB cell edge domain in a wild-type cotyledon epidermal cell. (c) MTs inclasp-1mutants undergo catastrophe on reaching cell edges, which lack CTBs. Shown are cotyledon epidermal cells. The scale bars represent 5 μm. Times are in seconds. (d) MT-edge catastrophe rates at GFP–CLASP-containing versus GFP–CLASP-free domains at the transverse and longitudinal edges of root epidermal division zone cells. Red indicates MT edge catastrophe, blue indicates MT edge passage (n=27 cells, 154 MTs). Figure 6b shows an example of MT persistence on encountering a CTB edge domain ( Supplementary Movie 6 ). In young clasp-1 leaf epidermal cells, which lack CTBs, the edge-induced MT catastrophe rate was 94.3±1.2% ( n =106 MTs, 19 cells), which is mildly elevated from the 84% rate observed at CTB-free domains in wild-type cells. Several examples of edge-induced catastrophes from a clasp-1 leaf cell are shown in Figure 6c ( Supplementary Movie 7 ). Figure 6: CLASP mitigates the barrier effect of sharp cell edges. ( a ) Percentage of MTs that undergo catastrophe on encounter of CTB versus CTB-free cell edges in young leaf epidermal cells. ( n =38 cells, 172 MTs; bars are mean percentages±s.e). Yellow brackets indicate CTBs, Red lines indicate CTB-free domains (using CTBs as proxies for GFP–CLASP domains.) ( b ) MT persistence on encountering a CTB cell edge domain in a wild-type cotyledon epidermal cell. ( c ) MTs in clasp-1 mutants undergo catastrophe on reaching cell edges, which lack CTBs. Shown are cotyledon epidermal cells. The scale bars represent 5 μm. Times are in seconds. ( d ) MT-edge catastrophe rates at GFP–CLASP-containing versus GFP–CLASP-free domains at the transverse and longitudinal edges of root epidermal division zone cells. Red indicates MT edge catastrophe, blue indicates MT edge passage ( n =27 cells, 154 MTs). Full size image In root cells, where we could more clearly co-visualize GFP–CLASP and RFP–TUB6, MTs encountering edge domains lacking GFP–CLASP were 13.8 fold more likely to undergo catastrophe compared with GFP–CLASP edge domains ( Fig. 6d ; Table 1 ; n =154 MTs, 27 cells). Table 1 Summary of cell-edge curvatures and edge catastrophe rates. Full size table These data are consistent with CLASP's role in locally promoting pause/rescue in vitro and in animal and yeast cells [35] , [36] , [37] . Effect of edge curvature on edge catastrophe Edge curvature-dependent catastrophe was also apparent in the older expanding cells ( Table 1 ). In elongating root cells, MTs encountering the semi-rounded, longitudinal edges underwent catastrophe for 26.2±4.8% of cases, compared with the 98.2% rate seen at the sharp transverse edges ( Fig. 6d ; n =50 cells, 141 MTs). In expanded leaf epidermal cells (in which CLASP content is low), MTs encountering edges underwent catastrophe in 65.7±4.4% of the cases, compared with the 84% rate seen in unexpanded cells ( Fig. 6d ; n =28 cells, 172 MTs). The higher catastrophe rates at rounded edges in expanded leaf cells compared with rounded edges in root cells is consistent with the edges in expanded leaf epidermal cells being sharper than the longitudinal edges of root cells (radius of curvature 2.5 versus 7.2 μm; Table 1 ). Furthermore, subdividing leaf cell edges into sharp (<3 μm) and round (>3 μm) reveals greater edge catastrophe rates in the sharp class, which further correlates edge curvature and catastrophe rates ( Table 1 ). Taken together, these data support a broad correlation between edge curvature and MT edge-induced catastrophe rates. Computer modelling cell edge effects on MT organization We next used computational simulations to test the hypothesis that MT organization can be controlled by modulating the ability of MTs to bypass the edges between cell faces. We simulated MTs migrating around the cortex using algorithms published previously [15] and parameters measured in this study ( Fig. 7 ) and previous ones [38] , [39] ( Supplementary Fig. S5 ; Methods). The simulations incorporated dynamic instability at the plus-end and continuous depolymerization at the minus-end, and MT–MT interactions through entrainment at low angles of collision and collision-induced catastrophe at high angles of collision. We approximated the cell as a cube and simulated the presence or absence of CLASP edge domains by modulating the ability of MTs to cross different edges. A MT encountering an edge undergoes edge-induced catastrophe with probability pcat i , where i =(Longitudinal, Transverse, Radial). The alternative outcome is growth of the MT around the edge. 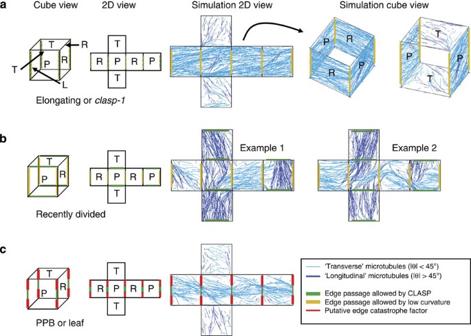Figure 7: Simulations of cortical MTs on a cube. These simulations use dynamic instability parameters measured from wild-type elongating cells at 21 °C reported in ref.39and a nucleation rate of 5 μm−2min−1. For all simulations, cells are shown schematically as 10×10 μm cubes, flattened cubes, and flattened cubes with MTs. Green edges represent CLASP domains, and have a low probability of edge-induced catastrophe. Golden edges represent low-curvature edges that also have low catastrophe (pcat=0.26). Non-coloured edges have a default high probability of inducing MT catastrophe. Transverse MTs (0–45°) are coloured light blue, and longitudinal MTs (45–90°) are coloured dark blue. For cell faces, T=transverse, R=radial, P=periclinal. For cell edges, T=Transverse, L=Longitudinal, R=Radial. SeeSupplementary Table S1for edge catastrophe values. (a) Elongating orclasp-1cells with transverse MT arrays are simulated by allowing MT passage on longitudinal edges only. (b) Recently divided cells with mixed MTs are simulated by decreasing the probability of edge-induced catastrophe specifically on the transverse edges, which is where CLASP protein is found. (c) Cells evocative of leaf epidermal cells or cells containing a PPB are simulated by allowing MTs to traverse the middle third of longitudinal edges (green). For simulating a PPB, red sectors highlight the possible sites of a hypothetical edge-based catastrophe factor. Figure 7: Simulations of cortical MTs on a cube. These simulations use dynamic instability parameters measured from wild-type elongating cells at 21 °C reported in ref. 39 and a nucleation rate of 5 μm −2 min −1 . For all simulations, cells are shown schematically as 10×10 μm cubes, flattened cubes, and flattened cubes with MTs. Green edges represent CLASP domains, and have a low probability of edge-induced catastrophe. Golden edges represent low-curvature edges that also have low catastrophe (pcat=0.26). Non-coloured edges have a default high probability of inducing MT catastrophe. Transverse MTs (0–45°) are coloured light blue, and longitudinal MTs (45–90°) are coloured dark blue. For cell faces, T=transverse, R=radial, P=periclinal. For cell edges, T=Transverse, L=Longitudinal, R=Radial. See Supplementary Table S1 for edge catastrophe values. ( a ) Elongating or clasp-1 cells with transverse MT arrays are simulated by allowing MT passage on longitudinal edges only. ( b ) Recently divided cells with mixed MTs are simulated by decreasing the probability of edge-induced catastrophe specifically on the transverse edges, which is where CLASP protein is found. ( c ) Cells evocative of leaf epidermal cells or cells containing a PPB are simulated by allowing MTs to traverse the middle third of longitudinal edges (green). For simulating a PPB, red sectors highlight the possible sites of a hypothetical edge-based catastrophe factor. Full size image For values of edge-induced catastrophe probabilities, we used our experimentally obtained values ( Table 1 ). Thus, for longitudinal edges, pcat longitudinal =0.26. For radial and transverse edges, we use the probabilities of edge-induced catastrophe measured in leaf cell edges at CTB-containing and CTB-free domains ( Fig. 7a ) as a proxy for edges with or without CLASP, respectively. These values are rounded to the nearest 5% and shown in Supplementary Table S1 . Simulations in which MTs easily bypass longitudinal edges, but undergo frequent catastrophe at transverse edges result in an array for which the dominant direction is transverse to the elongation axis ( Fig. 7a ), in agreement with simulations in Allard et al . [15] . This simulation represents elongating cells, which have low CLASP levels and cells of the clasp-1 mutant, which establish transverse MT arrays soon after division. In these simulations, MT arrays on the transverse faces self-organize in independent, random directions and have fewer MTs per unit area. Increasing the ability of MTs to grow around the transverse edges (modelling the observed localization and role of CLASP in recently divided cells) generated a large increase in longitudinally oriented MTs, resulting in a mixed array, containing both longitudinal and transverse MTs ( Fig. 7b ). This shows that decreasing the differential in MT edge pass-ability between edges can lead to less ordered MT arrays. Simulating a cell in which only the middle third of the longitudinal edges allows MT passage resulted in a transverse band of MTs running around the middle of the cell, which is evocative of PPBs and early leaf epidermal cells, which have non-uniform bundling within individual faces ( Fig. 7c ). Further permutations are included in the Methods section. How plant cells orient cortical MTs has remained enigmatic ever since 1963 when these cytoskeletal elements were first described [40] . Here we demonstrate, both by live imaging and computational modelling, that the intrinsic geometry of cells provides an external organizing cue that can bias the orientation of cortical MTs. Specifically, the sharp cell edges that are found in small boxy cell types, such as those in meristems and expanding leaves, present a physical barrier that, by impeding assembly of MTs growing into them, enriches for MTs running parallel to them. Importantly, it is the differential pass-ability of cell edges that provides a spatial cue for orienting cortical MTs. This is clearly illustrated in root tip cells, which have sharp transverse edges at the newly formed cross walls that act as barriers to MTs, and rounded longitudinal edges (derived from more distant divisions) that are more passable to MTs. Plants lacking CLASP reveal the default MT response to this geometric polarity cue: MTs orient parallel to the transverse edges, resulting in transverse arrays. To generate the mixed arrays present at the outer periclinal face of recently divided wild-type root tip cells, it is necessary to provide further MT stabilization by CLASP protein accumulation at the transverse edges. This reduces the catastrophe frequency nearly tenfold to enable incoming longitudinal MTs to grow around these sharp edges and form CTBs. In agreement with these data, when MTs on adjacent anticlinal faces enter the shared periclinal face from two disparate orientations, a criss-cross pattern is generated [1] . The randomized distribution of MTs in clasp-1 leaf epidermal cells eventually corrects itself when edges become rounded enough to allow MT passage, and MTs even achieve a hyperparallel organization because of increased cortex detachment and MT interactions [11] . Thus, an inherent bias toward MT parallelism is driven by self-organizational mechanisms. Interestingly, edge-induced MT depolymerization is reminiscent of previous observations of collision-induced catastrophe on encounter of one MT with another at large encounter angles [6] . Physical barriers that impede MT growth can increase the rate of MT catastrophe [34] , [41] , possibly by retarding MT growth while GTP hydrolysis continues, thereby depleting the GTP-cap [15] . Because curved MT growth requires extra bending energy in the MT lattice, curvature acts as a physical barrier that will locally increase the catastrophe frequency. This effect can be incorporated into the model by reducing the polymerization rate by an appropriate factor as outlined in the dimer-level model of Allard et al . [15] Given this curvature-sensitive growth, MTs growing towards a particular edge have a probability of edge-induced catastrophe that depends on the edge's curvature and MT-edge encounter angle. At first glance, the probability of catastrophe might be expected to have an increasing dependence on both curvature and angle. The problem, however, is quite subtle. A shallow angle of incidence means the MT will encounter a lower curvature but will be sustained over a longer path length. Depending on the relationship between curvature-induced and instantaneous catastrophe rate, an edge's catastrophe probability could hypothetically increase or decrease with varying angle of incidence. As dependence on angle-of-incidence has not been quantified experimentally or theoretically, in the present work, we use population averages of all MTs encountering a particular edge. CLASP has been reported to locally alter MT dynamics in yeast and animal cells by promoting MT rescue [36] , [42] . If this function is conserved in plants, CLASP could be counteracting the catastrophe-inducing influence of the edge's curvature. A schematic of CLASP-induced edge tolerance is shown in Supplementary Figure S6 . In the present study, we have not investigated the mechanism of CLASP edge targeting, but future work will address this. Stereotypical MTOCs, such as centrosomes in animal cells and spindle pole bodies in fungal cells, are discrete centres that act locally but influence cell-wide MT organization. By locally tethering MT minus ends, centrosomes ensure that MTs radiate from a central point, allowing plus-ends to interact with the cortex. We propose that the plant cell edge also fits the criteria of a MTOC: by locally inducing catastrophe or allowing passage of MT plus-ends at specific sites along the cell edges, cell-wide MT organization is generated. We also propose that CLASP works in concert with the cell edge to act as a 'tuneable MTOC'. By modulating the location and degree of catastrophe, CLASP is able to generate cell-wide ordering of MTs. The data suggest a molecular mechanism for the previous observation of MT foci at cell edges in the fern Azolla [31] , [43] . CLASP also functions in elongating cells, as indicated by its association with transverse MTs in these cells and the significantly reduced density of MT populations in the clasp-1 mutant [30] . It is nonetheless not required for generating transverse order. Indeed, the precocious establishment of transverse MT arrays in clasp-1 and the reduction in CLASP protein levels as cells enter the root elongation zone suggest that CLASP-recruiting factors at sharp transverse edges are required to overcome a strong inherent bias toward transverse arrangement. Given that GFP–CLASP edge domains are intersected by CTBs, it is possible these bundles provide protective tracks for incoming MTs, thereby indirectly allowing edge passage, instead of a direct CLASP-based stabilization. Indeed we observed many instances of MTs encountering TBs, becoming entrained with them, and continuing growth around the edge, consistent with dynamic turnover of MTs within bundles [2] , [44] . MT-bundle entrainment was also occasionally apparent in the case of TBs within mature leaf epidermal cells (where CLASP is low or absent). As documented in our current study, MTs encountering GFP–CLASP-free edges underwent frequent catastrophe, yet GFP–CLASP did not accumulate. In other cases, however, GFP–CLASP appearance at cell edges coincided with arrival of incoming MTs. Therefore, CLASP recruiting factors might reside at select edge domains, where, by complexing with a CLASP-coated MT (or possibly plus-end-associated CLASP), they can allow edge passage. This CLASP-based stabilization of select 'pioneer' MTs could also establish the initial MT tracks for extra MTs during CTB formation. Leaf epidermal cells attain their distinctive interdigitated shape as a result of non-uniform MT bundling around the anticlinal edges [32] , [33] . This mechanism is thought to be distinct from that in other cell types, in which MTs attain a more uniform organization on all faces. On the basis of our data, however, we postulate that all cases of non-uniform MT bundling about the anticlinal faces (such as PPBs and tracheary element MT bands) are manifestations of a fundamental mechanism that is present in all young plant cells. Plant materials and growth conditions Arabidopsis thaliana Columbia ecotype plants were grown in continuous light conditions on vertical agar plates containing Hoagland's medium. Young expanding cotyledon cells were imaged at 3–4 days. Root tips were used for dividing and expanding root cells. Cloning For the pCLASP:GFP–CLASP construct, DNA was amplified from 2,040 bp upstream up to the ATG start codon of the CLASP gene (At2g20190), and cloned into the HindIII/Sal1p sites of a modified pCAMBIA1300 vector containing smrsGFP followed by a 10×alanine linker, followed by the full coding sequence of the CLASP gene. Primers were fwd 5′-atttctttgcttccttctc-3′, and rev 5′-tttttaccaaaccaccgacgga-3′. For pUBQ1:mRFP–TUB6, 2,322 bp upstream sequence from the Arabidopsis Ubiquitin 1 gene was cloned into the HindIII/Sal1p sites of a modified pCAMBIA1300 vector containing mRFP–TUB6. This reporter is far superior to previous 35S promoter driven RFP–TUB6 because it is expressed throughout the root and aerial tissues. Furthermore, its low expression in lateral root cap cells relative to the underlying tissues allows clear observation of epidermal division zone and elongation zone cells. Immunofluorescence and root squashing Immunofluorescence was performed as in Ambrose et al . [30] Arabidopsis seedlings grown on vertical agar plates were fixed for 1 h (4% formaldehyde (freshly prepared from paraformaldehyde), 50 mM Pipes pH 6.9, 5 mM EGTA, 1 mM MgSO 4 , 1% glycerol), rinsed, and digested with cell-wall-degrading enzymes (0.5% cellulose, 0.05% pectolyase, 0.5% Triton X-100) for 15 min. Specimens were then treated with 3% bovine serum albumin for 1 h in a humidity chamber, rinsed, and detergent-extracted for 20 min in 0.5% Triton X-100 before incubation in fluorescein isothiocyanate-conjugated DMA1 anti-tubulin antibody (1:75 dilution; Sigma) for 1.5 h. Specimens were mounted in Citifluor AF1 anti-fade agent. To illustrate the distribution of GFP–CLASP within individual cells, roots were fixed and squashed onto slides to separate cells. GFP–CLASP-expressing plants were fixed using a fixation regime that preserved GFP fluorescence. Subsequent to fixing, root tips were squashed onto poly- L -Lysine-coated slides to foster separation and adherence of cells. Microscopy and image analysis Images were acquired on a Zeiss Pascal scanning confocal microscope, or with a Perkin-Elmer spinning disk microscope. Images were processed using imageJ software ( http://rsb.info.nih.gov/ij/ ), and figures were assembled using Corel Draw software. MT arrays were classified as transverse, longitudinal, or mixed relative to the long axis of the root on a cell by cell basis. If over 90% of visible MTs in the cell fit a given orientation, that orientation was assigned. Transverse MTs were oriented within 0–30° of the transverse axis, longitudinal MTs were 60–90°, and cells designated mixed contained populations of both directions in similar proportions, or an abundance of MTs in oblique orientations (30–60°). For analysis of RFP–TUB6 in root tissues, we drove expression under the Ubiquitin 1 promoter, which, unlike the 35S promoter-driven RFP–TUB6, enabled the clear visualization of MTs in all root tissues. Computer simulations We used a modified version of the simulation described in Allard et al . [15] with kinetic parameters taken from wild type (WT) at 31 °C and interaction parameters including both entrainment and collision-induced catastrophe. We simulated uniform nucleation at random angles at a rate of 5 min −1 m −1 . Instead of the two-dimensional geometry we described in Allard et al . [15] , we simulated on six faces of a cube. When the plus-end of a MT is incident on an edge, two outcomes are possible: with probability p i , the plus-end undergoes catastrophe; or, with probability (1- p i ), the MT becomes split into two segments, with one segment on the connecting face at an equal angle relative to the edge. Here i is the class of edge (transverse, longitudinal or radial). Edge catastrophe probabilities for all simulations were taken from quantitative measurements performed in this study ( Table 1 ), and are summarized in Supplementary Table S1 . Snapshots were taken 120 min after initiation of assembly in an initially empty cube. Simulations were carried out on WestGrid (Compute/Calcul Canada). Sensitivity of simulations The simulations presented in Figure 6 use dynamic instability parameters measured from WT elongating cells at 21 °C reported in Kawamura and Wasteneys [39] and a nucleation rate of 5 μm −2 min −1 . This nucleation rate reproduces a density of MTs that closely approximates the density in observed cortical MT arrays. We obtained similar results using dynamic instability parameters from WT elongating cells at 31 °C (ref. 39 ), shown in Supplementary Figure S5a, and parameters from WT division phase cells reported in Vos et al . [38] with a nucleation rate of 0.2 μm −2 min −1 , shown in Supplementary Figure S5b . In the case of low nucleation rates, the MT pattern is the same but with lower MT density. These figures demonstrate that our results are robust to changes in nucleation rate and independent of whether the dynamic instability parameters are in the 'bounded' or 'unbounded' regime (for details see refs 15 , 45 ) because the WT at 21 °C parameters are in the unbounded regime. Note that for unbounded parameters, the mean length and number of MTs increase gradually as the simulation continues, whereas the array ordering, described by an order parameter [14] , [15] , saturates at a steady-state value. We also observe very similar MT patterns for the dynamic instability parameters described in Shaw et al . [2] and Dixit and Cyr [6] and nucleation rates ranging from 0.2 to 10 μm −2 min −1 (data not shown). Sensitivity of simulations to changes in edge catastrophe rates We determined that the upper limit of curvature that can still allow transverse arrays to form is an ∼ 60% catastrophe rate ( Supplementary Fig. S7a ). Catastrophe rates above this were unable to generate cell-wide order. Simulating CLASP at transverse as well as radial edges (pcat transverse =0.1, and pcat radial =0.1) generated random arrays ( Supplementary Fig. S7b ). How to cite this article: Ambrose, C. et al . A CLASP-modulated cell edge barrier mechanism drives cell-wide cortical microtubule organization in Arabidopsis. Nat. Commun. 2:430 doi: 10.1038/ncomms1444 (2011).